Direct-current voltages in (Ga,Mn)As structures induced by ferromagnetic resonance Spin pumping is the phenomenon that magnetization precession in a ferromagnetic layer under ferromagnetic resonance produces a pure spin current in an adjacent non-magnetic layer. The pure spin current is converted to a charge current by the spin–orbit interaction, and produces a d.c. voltage in the non-magnetic layer, which is called the inverse spin Hall effect. The combination of spin pumping and inverse spin Hall effect has been utilized to determine the spin Hall angle of the non-magnetic layer in various ferromagnetic/non-magnetic systems. Magnetization dynamics of ferromagnetic resonance also produces d.c. voltage in the ferromagnetic layer through galvanomagnetic effects. Here we show a method to separate voltages of different origins using (Ga,Mn)As/p-GaAs as a model system, where sizable galvanomagnetic effects are present. Neglecting the galvanomagnetic effects can lead to an overestimate of the spin Hall angle by factor of 8, indicating that separating the d.c. voltages of different origins is critical. The introduction of spin polarization to non-magnetic semiconductors is an important step for realizing novel spintronics devices [1] . So far, various schemes have been demonstrated to generate and detect spin current in non-magnetic semiconductors, which include electrical and optical means [2] , [3] , [4] , [5] , [6] , [7] , [8] , [9] , [10] . Spin pumping is known as a method to generate a pure spin current without a net flow of charge current in non-magnetic materials adjacent to a ferromagnetic layer under ferromagnetic resonance (FMR). When the FMR condition for the ferromagnetic layer is fulfilled, precession of magnetization creates excess spin-polarized carriers in the ferromagnetic layer due to damping caused by the exchange interaction between magnetic spins and carriers [11] , [12] . The excess spin polarization of carriers in the ferromagnetic layer penetrates into the adjacent non-magnetic layer, which generates spin current in the vicinity of the interface but no charge current under zero bias. The pure spin current can be detected electrically as a d.c. electromotive force induced by the inverse spin Hall effect (ISHE), which converts spin current J s to charge current J c through the spin–orbit interaction: J c θ SHE J s × σ , where θ SHE is the spin Hall angle and σ is the spin polarization unit vector [13] , [14] . Thus, by measuring the d.c. electromotive force, one can determine the value of θ SHE . Spin injection and detection based on spin pumping and the ISHE have been applied to a variety of material systems [13] , [14] , [15] , [16] , [17] , [18] , [19] , [20] , [21] , [22] , [23] . Recent work showed that it may be a promising tool for the generation and investigation of spin current in semiconducting materials, such as Si (refs 16 , 17 ), Ge (refs 18 , 19 ) and GaAs with n-type as well as p-type conduction [20] . Magnetization dynamics under FMR also produces d.c. voltage in the ferromagnetic layer through galvanomagnetic effects, that is, anisotropic magnetoresistance and anomalous Hall effect (AHE) [24] , [25] , [26] . These effects have often been neglected in the quantitative analyses on the observed d.c. voltage generated in a non-magnetic layer next to a ferromagnetic layer under FMR; the non-negligible contribution of these effects was pointed out only recently [22] , [23] , [27] . It is known that a ferromagnetic (Ga,Mn)As, which can be grown seamlessly on GaAs [28] , shows sizable galvanomagnetic effects [29] , [30] , and thus we expect that (Ga,Mn)As/p-GaAs bilayer structure is a suitable system to investigate the d.c. voltage observed under FMR. In this work, we systematically investigate d.c. voltages generated in a p-GaAs layer beneath an epitaxially grown (Ga,Mn)As layer under FMR, which are measured as functions of the magnitude of external magnetic field, magnetic field direction, microwave power and temperature. The results are analyzed by a phenomenological transport model in combination with the Landau–Lifshits–Gilbert (LLG) equation, which shows that the observed d.c. voltage is induced by the ISHE in p-GaAs accompanied by spin pumping as well as transverse galvanomagnetic effects, that is, the planar Hall effect (PHE, which is the transverse component of anisotropic magnetoresistance, and not a genuine Hall effect in the strict sense) and AHE in (Ga,Mn)As. We show both the ISHE and PHE result in a symmetric lineshape of d.c. voltage in their magnetic field dependence, while AHE has an anti-symmetric lineshape. The analysis of the magnetic field angle dependence of d.c. voltages enables us to deduce the ratio of the d.c. voltage by the ISHE to that by the PHE, because the voltages brought about by the two effects have different angle dependence. This analysis shows that the magnitude of d.c. voltage induced by the ISHE is about eight times smaller than that by the PHE. The spin Hall angle of p-GaAs is determined to be 0.006 from the magnitude of d.c. voltage induced by the ISHE, which is also about eight times smaller than that obtained by neglecting the presence of the PHE, indicating the importance of separating the d.c. voltages of different origins. Sample A bilayer structure studied here consists of a 20-nm Ga 0.935 Mn 0.065 As and a 20-nm p-GaAs on a semi-insulating GaAs (001) substrate with a 100-nm undoped GaAs buffer layer all grown epitaxially by molecular beam epitaxy (see Methods, we also grow a single (Ga,Mn)As for reference). The p-GaAs layer is Be-doped GaAs with hole concentration p of 9.5 × 10 18 cm −3 . We cleave the grown epitaxial wafer into a 1 × 3 mm 2 piece with a longer side along the [110] orientation. The top (Ga,Mn)As layer except for a central area with 1 × 2 mm 2 is etched away, and two In ohmic contacts are formed at the two ends of bare GaAs:Be surface by annealing at 250 °C for 30 min. This heat treatment increases the Curie temperature T C of (Ga,Mn)As from 79 K to 118 K (ref. 31 ). The schematic of the sample is shown in Fig. 1a . 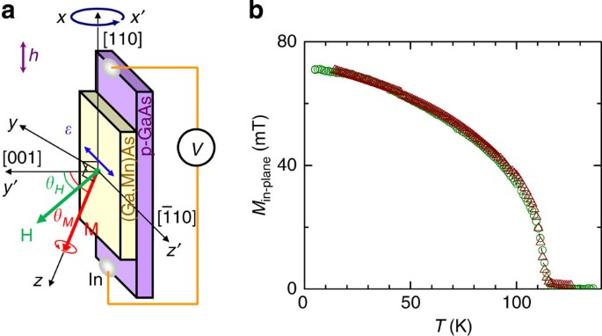Figure 1: d.c. voltage measurements and temperature dependence of magnetization. (a) Schematic of measurement configuration for d.c. voltage, which is measured simultaneously with FMR spectrum. The Cartesian coordinate systems used in analyses are also presented. (b) The temperatureTdependence of in-plane magnetization for (Ga,Mn)As/p-GaAs (triangles) as well as (Ga,Mn)As/undoped GaAs (circles). We confirm that linear current–voltage characteristics between the ohmic contacts and (Ga,Mn)As/p-GaAs junction at reduced temperature T of 30 K. Figure 1b compares the temperature T dependence of magnetization M of (Ga,Mn)As on p-GaAs with that on undoped GaAs (reference sample) after the same heat treatment, in which one can see that both (Ga,Mn)As layers have virtually identical magnetic properties. Figure 1: d.c. voltage measurements and temperature dependence of magnetization. ( a ) Schematic of measurement configuration for d.c. voltage, which is measured simultaneously with FMR spectrum. The Cartesian coordinate systems used in analyses are also presented. ( b ) The temperature T dependence of in-plane magnetization for (Ga,Mn)As/p-GaAs (triangles) as well as (Ga,Mn)As/undoped GaAs (circles). Full size image FMR spectra and d.c. voltages The sample is mounted on a quartz sample rod and put in a TE 011 microwave cavity, in which a magnetic (electric) field of the microwave is maximized (minimized). Microwave with frequency f 0 =9.0 GHz is introduced to the cavity in a cryostat. Twisted Cu wires are bonded to the ohmic contacts and are connected to a d.c. voltmeter. We measure FMR (microwave absorption) spectrum and d.c. voltage V between the two ohmic contacts simultaneously by sweeping the magnitude of an external magnetic field H . The ac modulation field H ac (1 mT, 100 kHz) parallel to H is superimposed to obtain FMR spectrum in its derivative form. To measure the angle ( θ H between H and [001] orientation) dependence of spectra, the sample is rotated about [110] axis, while keeping the (110) plane parallel to H ( Fig. 1a ). The same measurements are done for (Ga,Mn)As/undoped GaAs reference sample with two In ohmic contacts at the two edges of the (Ga,Mn)As surface ( Supplementary Fig. S1b ). 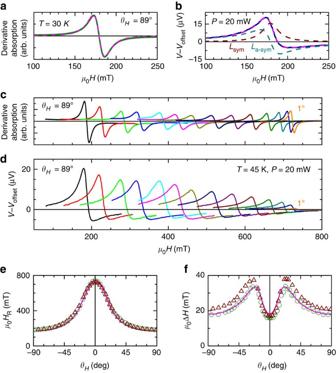Figure 2: FMR spectra and d.c. voltages. Typical spectrum of (a) FMR and (b) d.c. voltageVobtained at temperatureT=30 K and magnetic field angleθH=89o, where offset voltageVoffsetis subtracted. Solid lines are experimental results and dashed lines are fitting. In panelb, symmetric and anti-symmetric components of fitting are also shown by dashed lines. TheθHdependence of (c) FMR spectra and (d)V–Voffsetobtained atT=45 K and microwave powerP=20 mW. TheθHdependence of (e) FMR resonant fieldsHRand (f) linewidths ΔHof (Ga,Mn)As/p-GaAs (triangles) as well as (Ga,Mn)As/undoped GaAs (circles). Solid lines show the fitting results. arb. units, arbitrary units. Figure 2 shows a typical result of (a) FMR spectrum and (b) V curve (offset voltage V offset is subtracted) under microwave power P =20 mW at T =30 K and θ H =89 o . The V offset is due to electromagnetic induction by the application of H ac . One can see a characteristic V signal in the vicinity of ferromagnetic resonant field H R . To describe the lineshapes of spectra, we introduce symmetric ( L sym =Δ H 2 /[4( H − H R ) 2 +Δ H 2 ]) and anti-symmetric Lorentzian ( L a-sym =−4Δ H ( H − H R )/[4( H − H R ) 2 +Δ H 2 ]), where H =| H | and Δ H is the linewidth (FWHM) [14] , [32] . As shown by dashed lines in Fig. 2a , the FMR absorption spectrum ( Fig. 2a ) is fitted well by −(2 I /πΔ H )d L sym /d H , where I is the absorption coefficient [33] , and V − V offset ( Fig. 2b ) is fitted well by the sum of V sym L sym and V a-sym L a-sym where V sym and V a-sym are the magnitudes of symmetric and anti-symmetric voltage components. The fits show that the FMR spectrum and two components (symmetric and anti-symmetric components) of the measured d.c. voltage have identical H R as well as identical Δ H , indicating a strong correlation between FMR in (Ga,Mn)As and V in p-GaAs. Fig. 2c show FMR spectra and V curves as a function of θ H measured at T =45 K and P =20 mW. The θ H dependence of H R and Δ H obtained from FMR spectra is summarized for (Ga,Mn)As/p-GaAs and (Ga,Mn)As/undoped GaAs in Fig. 2e , respectively. While H R is identical for both samples, a larger Δ H for (Ga,Mn)As/p-GaAs is observed. This increase in Δ H is known to be caused by spin pumping, which produces additional damping by the diffusion of spin angular momentum into the adjacent layer [11] . (The θ H dependence of H R and Δ H for (Ga,Mn)As/undoped GaAs can be explained well by conventional analyses, which are shown in Fig. 2e by solid lines [34] , [35] , [36] , see Supplementary Note 1 ). Figure 2: FMR spectra and d.c. voltages. Typical spectrum of ( a ) FMR and ( b ) d.c. voltage V obtained at temperature T =30 K and magnetic field angle θ H =89 o , where offset voltage V offset is subtracted. Solid lines are experimental results and dashed lines are fitting. In panel b , symmetric and anti-symmetric components of fitting are also shown by dashed lines. The θ H dependence of ( c ) FMR spectra and ( d ) V – V offset obtained at T =45 K and microwave power P =20 mW. The θ H dependence of ( e ) FMR resonant fields H R and ( f ) linewidths Δ H of (Ga,Mn)As/p-GaAs (triangles) as well as (Ga,Mn)As/undoped GaAs (circles). Solid lines show the fitting results. arb. units, arbitrary units. 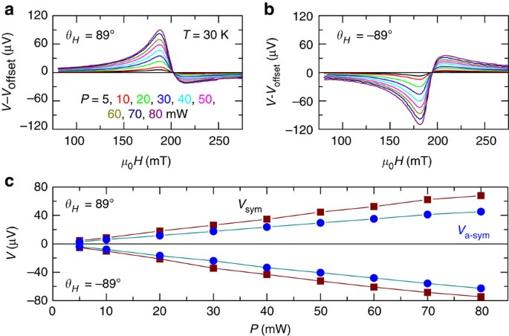Figure 3: Microwave power dependence of d.c. voltages. (a) Magnetic field angleθH=89oand (b)θH=−89oat temperatureT=30 K. (c) Microwave power dependence of magnitudes of symmetric (Vsym, squares) and anti-symmetric (Va-sym, circles) components of d.c. voltages forθH=−89oand 89oat 30 K. Full size image Microwave power dependence of d.c. voltages Figure 3a shows V − V offset as a function of P at 30 K, and at θ H =89 o and −89 o , respectively. The signal shows an opposite polarity with opposite θ H . The V sym and V a-sym obtained from the fit increase in proportion to P as shown in Fig. 3c , showing that the both components are related to FMR. Figure 3: Microwave power dependence of d.c. voltages. 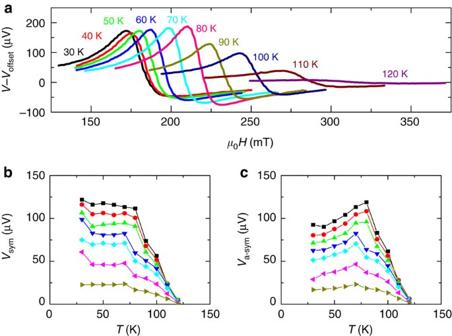Figure 4: Temperature dependence of d.c. voltages. (a) Spectra obtained at microwave powerP=100 mW and magnetic field angleθH=89oas a function of temperatureT. TheTdependence of (b) symmetric d.c. voltageVsymand (c) anti-symmetric d.c. voltageVa-symas a function ofPranging from 20–100 mW (black 100 mW, red 90 mW, green 80 mW, dark blue 70 mW, light blue 60 mW, pink 40 mW, olive green 20 mW). ( a ) Magnetic field angle θ H =89 o and ( b ) θ H =−89 o at temperature T =30 K. ( c ) Microwave power dependence of magnitudes of symmetric ( V sym , squares) and anti-symmetric ( V a-sym , circles) components of d.c. voltages for θ H =−89 o and 89 o at 30 K. Full size image Temperature dependence of d.c. voltages Figure 4a shows the T dependence of V − V offset measured under P =100 mW at θ H =89 o . The Δ H increases above 80 K, which is consistent with previous FMR results on (Ga,Mn)As [37] . The T dependence of V sym and V a-sym at various P from 20–100 mW is presented in Fig. 4b , respectively, in which the signals decrease to zero as T approaches T C , showing that the signals are indeed related to the magnetization dynamics in (Ga,Mn)As. The temperature at which FMR signal disappears is in good agreement with T C determined by magnetization measurements, indicating that heating caused by microwave absorption is negligible. By changing the measurement configuration, we rule out possible contribution from transverse thermoelectric effect (Nernst-Ettingshausen effect) to V in the present structure ( Supplementary Note 5 ). The magnitude of V sym shows a monotonic decrease with the increase of T , while that of V a-sym does not, suggesting that the two signals have different origins. Figure 4: Temperature dependence of d.c. voltages. ( a ) Spectra obtained at microwave power P =100 mW and magnetic field angle θ H =89 o as a function of temperature T . The T dependence of ( b ) symmetric d.c. voltage V sym and ( c ) anti-symmetric d.c. voltage V a-sym as a function of P ranging from 20–100 mW (black 100 mW, red 90 mW, green 80 mW, dark blue 70 mW, light blue 60 mW, pink 40 mW, olive green 20 mW). Full size image There are three possible origins of the observed d.c. voltage induced by magnetization dynamics; one is the ISHE [14] , and the other two are transverse galvanomagnetic effects, i.e., PHE and AHE [38] . We use the LLG equation, d M /d t =− γ M × μ 0 H eff +( α /| M |) M × d M /d t , to describe the magnetization dynamics, where M is the magnetization vector, d M /d t its time derivative, γ the gyromagnetic ratio, μ 0 the permeability in vacuum and α the damping constant [39] . The first and second terms in the LLG equation correspond to precessional and damping torques, respectively. We use a Cartesian coordinate system with x along [110] and z along the precession axis of M as shown in Fig. 1a , and thus M =( m x e iωt , m y e iωt , M z ), where ω is the angular frequency of precession. The effective magnetic field vector H eff is the sum of an external magnetic field, magnetic anisotropy fields, their dynamical components, and microwave field h = e i ω 0 t ( h , 0, 0) with ω 0 =2 πf 0 . By solving the LLG equation, one can calculate the H dependence of complex susceptibility χ as well as the real (Re) and imaginary (Im) parts of m x and m y : Re( m x ), Im( m x ), Re( m y ), and Im( m y ) (see Supplementary Notes 1, 2 and 3 ). The ISHE signal V ISHE in p-GaAs results from the pure spin current with spin polarization along in-plane z ′ direction ([ ] orientation) generated by spin pumping, which flows perpendicular direction to the interface between (Ga,Mn)As and p-GaAs. Because the spin current induced by spin pumping is proportional to the damping term in the LLG equation, V ISHE is expected to be proportional to the time averaged z ′ projection of the damping term [11] , [40] , V ISHE ( αω / M z )[Im( m x )Re( m y )−Re( m x )Im( m y )]sin θ M , where θ M is the angle between M and [001] orientation (the overscore denotes the time average). When the sample size is finite, electric field ε of microwave along z ′ direction ( Fig. 1a ) may generate the PHE and AHE signals ( V PHE and V AHE ) in (Ga,Mn)As. We obtain V PHE εM z Re( m x )sin θ M and V AHE εM z Re( m y )sin θ M , where x || x ′. 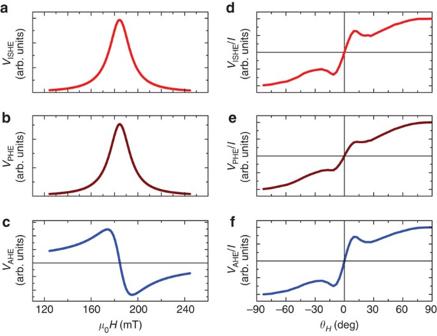Figure 5: Calculated lineshapes and magnetic field angle dependence of d.c. voltages. In calculation, experimentally obtained parameters are utilized (Supplementary Note 1). (a–c) Lineshapes of d.c. voltages induced by the ISHE (VISHE), PHE (VPHE) and AHE (VAHE) under in-plane magnetic field. (d–f) Out-of-plane field angleθHdependences ofVISHE,VAHEandVPHE, which are normalized by microwave absorption coefficientI. arb. units, arbitrary units. Figure 5 shows the calculated lineshapes and θ H dependences of ISHE, PHE and AHE, which indicates that V ISHE and V PHE have symmetric lineshape, whereas V AHE has anti-symmetric lineshape, and that the three signals have the same linewidth. Although it is hard to distinguish the ISHE from the PHE in each spectrum due to the same symmetry and linewidth, the difference in θ H dependence ( Fig. 5d ) allows us to separate the components of the ISHE and PHE from V sym . Figure 5: Calculated lineshapes and magnetic field angle dependence of d.c. voltages. In calculation, experimentally obtained parameters are utilized ( Supplementary Note 1 ). ( a – c ) Lineshapes of d.c. voltages induced by the ISHE ( V ISHE ), PHE ( V PHE ) and AHE ( V AHE ) under in-plane magnetic field. ( d – f ) Out-of-plane field angle θ H dependences of V ISHE , V AHE and V PHE , which are normalized by microwave absorption coefficient I . arb. units, arbitrary units. Full size image In Fig. 6a , we show the θ H dependence of normalized V sym / I as well as the fit, which is sum of calculated V ISHE / I and V PHE / I curves, and the ratio of the two signals is adopted as a fitting parameter. The fitting reproduces the θ H dependence of V sym / I well, and shows that the contributions to V sym from the ISHE and PHE are 11.8% and 88.2%, respectively. 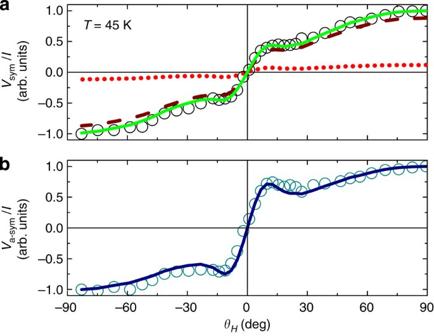Figure 6: Angle dependence of d.c. voltage. Open circles denote the d.c. voltage obtained at 45 K. Magnetic field angleθHdependence of (a) symmetric componentVsymand (b) anti-symmetric componentVa-symof d.c. voltage, normalized by microwave absorption coefficientI. Dotted and dashed lines in panelashow theθHdependence of d.c. voltages induced by the inverse spin Hall effectVISHE/Iand planar Hall effectVPHE/I, where the ratio of the magnitudes ofVISHEandVPHEis adjusted to reproduce the experimental result. Solid line represents total contributions,VISHE/I+VPHE/I. Solid line inbshows theθHdependence of d.c. voltage induced by the AHEVAHEnormalized byI. arb. units, arbitrary units. Figure 6b shows the θ H dependence of normalized V a-sym / I and the calculated AHE curve, which shows that the θ H dependence of V a-sym can be described well by V AHE . Moreover, non-monotonic T dependence of V a-sym in Fig. 4c supports that the origin of V a-sym is the AHE, because similar non-monotonic T dependence of the anomalous Hall resistance is observed in d.c. transport measurements using a Hall bar. The observed comparable magnitudes of V sym and V a-sym in d.c. voltages ( Figs 3c and 4b ) agree with what we expect from the amplitudes of planar Hall and anomalous Hall resistances determined by d.c. transport measurements ( Supplementary Note 4 ). Figure 6: Angle dependence of d.c. voltage. Open circles denote the d.c. voltage obtained at 45 K. Magnetic field angle θ H dependence of ( a ) symmetric component V sym and ( b ) anti-symmetric component V a-sym of d.c. voltage, normalized by microwave absorption coefficient I . Dotted and dashed lines in panel a show the θ H dependence of d.c. voltages induced by the inverse spin Hall effect V ISHE / I and planar Hall effect V PHE / I , where the ratio of the magnitudes of V ISHE and V PHE is adjusted to reproduce the experimental result. Solid line represents total contributions, V ISHE / I + V PHE / I . Solid line in b shows the θ H dependence of d.c. voltage induced by the AHE V AHE normalized by I . arb. units, arbitrary units. Full size image From V sym =15 μV at T =45 K and P =20 mW, V ISHE is calculated to be 1.77 V. By using this value, the spin Hall angle of p-GaAs is obtained to be 0.006 ( Supplementary Note 6 ). If the entire symmetric component ( V sym =15.0 μV) were treated as the ISHE signal, the spin Hall angle would have been θ SHE =0.05, which is comparable with heavy metals (Liu et al. [41] and references therein). We also measure d.c. voltage of a 10-nm-thick permalloy (Py) film deposited on thermally oxidized Si substrate, which shows that Py also generates symmetric and anti-symmetric voltages induced by galvanomagnetic effects (not shown), although the magnitudes of them are sensitive to Ni-Fe composition (Py has large PHE and small AHE) [42] . As Py-based structures is one of the most investigated systems for spin pumping and ISHE [14] , [16] , [17] , [18] , [20] , [21] , [22] , [23] , our approach used here is useful for systems other than the (Ga,Mn)As-based one. In summary, we have demonstrated spin injection from (Ga,Mn)As into p-GaAs by means of spin pumping and its detection by the inverse spin Hall effect. While the PHE produces the same symmetric spectral lineshape as that of the inverse spin Hall effect, we have shown that the two can be separated by measuring the angle dependence of the signal. This allows us to determine the spin Hall angle of p-GaAs ( p =9.5 × 10 18 cm −3 ) as 0.006. The present study shows that one needs to take sufficient care to convert d.c. voltages to the inverse spin Hall effect and thus to the spin Hall angle of the non-magnetic layer, indicating the critical importance of separating the inverse spin Hall effect from galvanomagnetic effects. Sample preparation (Ga,Mn)As (20 nm, Mn composition x =0.065)/GaAs:Be (20 nm, hole concentration p =9.5 × 10 18 cm −3 ) bilayer structure is grown on semi-insulating GaAs (001) substrate by molecular beam epitaxy through a GaAs (100 nm) buffer layer. The growth temperature is 560 o C for GaAs buffer and GaAs:Be and 250 °C for (Ga,Mn)As. During growth, V/III beam equivalent pressure ratio is kept at 8. The carrier concentration of GaAs:Be is calibrated by room-temperature Hall measurements on separately prepared 1-μm-thick GaAs:Be layers. The thickness of GaAs:Be (20 nm) is a few times thicker than a surface-depletion layer of p-GaAs with p ~;10 19 cm −3 . The wafer is cleaved into a piece with lateral dimension of 1 × 3 mm 2 and then the two edge regions of top (Ga,Mn)As are removed by wet etching to pattern 1 × 2 mm 2 rectangular (Ga,Mn)As mesa. The etching depth is ~;25 nm, which is confirmed by atomic force microscopy. The samples is annealed at 250 ° C for 30 min in air, to form two In ohmic contacts on exposed surface of GaAs:Be. A reference sample without GaAs:Be layer is also prepared by virtually identical growth and annealing conditions. How to cite this article : Chen, L. et al. Direct-current voltages in (Ga,Mn) As structures induced by ferromagnetic resonance. Nat. Commun. 4:2055 doi: 10.1038/ncomms3055 (2013).